Exhaustion of nucleus pulposus progenitor cells with ageing and degeneration of the intervertebral disc Despite the high prevalence of intervertebral disc disease, little is known about changes in intervertebral disc cells and their regenerative potential with ageing and intervertebral disc degeneration. Here we identify populations of progenitor cells that are Tie2 positive (Tie2 + ) and disialoganglioside 2 positive (GD2 + ), in the nucleus pulposus from mice and humans. These cells form spheroid colonies that express type II collagen and aggrecan. They are clonally multipotent and differentiated into mesenchymal lineages and induced reorganization of nucleus pulposus tissue when transplanted into non-obese diabetic/severe combined immunodeficient mice. The frequency of Tie2 + cells in tissues from patients decreases markedly with age and degeneration of the intervertebral disc, suggesting exhaustion of their capacity for regeneration. However, progenitor cells (Tie2 + GD2 + ) can be induced from their precursor cells (Tie2 + GD2 − ) under simple culture conditions. Moreover, angiopoietin-1, a ligand of Tie2, is crucial for the survival of nucleus pulposus cells. Our results offer insights for regenerative therapy and a new diagnostic standard. Degeneration of the intervertebral disc (IVD) is a significant cause of back pain and has a large economic burden [1] . By creating instability, IVD degeneration is also a trigger for most spinal diseases and can lead to secondary spinal deformity and spinal canal stenosis [2] . The IVD is composed of an inner nucleus pulposus (NP) surrounded by the annulus fibrosus (AF) and thin hyaline cartilaginous end-plates between the IVD and the adjacent vertebral bodies. The gelatinous NP is an avascular tissue containing extracellular matrix (ECM) comprising highly hydrated proteoglycan and collagen [3] . Although loss of ECM-producing cells accounts for IVD degeneration [4] , the pathogenesis of IVD degeneration is largely unknown and there are no effective therapies. The IVD undergoes degenerative changes earlier in life than do other tissues of major organ systems that comprise long-lived cells that are normally replaced infrequently [5] , [6] , [7] . The functional ability of IVD cells changes over time during the process of degeneration and ageing. The cells respond to the changes induced by environmental damage and stress by entering a state of cell senescence [8] , during which the ECM surrounding such cells and neighbouring cells may be altered. Under these circumstances, the resilience of the IVD cell population might be ensured if the relevant stem cell populations could give rise to differentiated progeny over a person’s lifetime. However, apart from a heterogeneous cell population derived from degenerate human IVD, which can differentiate into mesenchymal lineages [9] , [10] , [11] , no single-cell progenitors have been identified in NP tissue. To identify NP stem and progenitor cells, we began with a colony-forming assay (CFA) using methylcellulose semi-solid medium, which was established to evaluate haematopoietic or endothelial stem/progenitor cells [12] , [13] and has been used to identify tissue-specific stem/progenitor cells from various organs [14] , [15] . We sorted human and mouse NP cells using various surface markers and then scored their ability to form colonies. Following this prescreening, cells were evaluated for clonogenicity in vitro and for multipotency and self-renewal ability in vivo . Finally, we identified progenitor cells in populations purified from adult mouse (m) and human (h) NP cells using two markers: the tyrosine kinase receptor Tie2 and disialoganglioside 2 (GD2). Our findings demonstrate an important role for angiopoietin-1, a ligand of Tie2, in maintaining these progenitor cells and protecting NP cells from apoptosis. The present work was undertaken to explore the hypothesis that the frequency of these progenitor cells in hNP tissues correlates with the clinical extent of IVD degeneration and ageing. Surface markers to select putative progenitor cells To find clues to the identity of the progenitor cells in the mNP, we evaluated NP cells from tail IVDs of 8- to 10-week-old C57BL/6 mice in CFA in methylcellulose medium. After 10 days, adhesive fibroblastic colonies and spheroid colonies were observed. We named these two types of colonies mNP colony-forming units-fibroblastic (mNP-CFU-F) and mNP colony-forming units-spherical (mNP-CFU-S), respectively. Both types of colonies were retrieved from the medium without enzymatic digestion and were visualized with immunocytochemical staining. mNP-CFU-S were strongly positive for type II collagen and aggrecan, whereas mNP-CFU-F were predominantly negative. Therefore, mNP-CFU-S were considered to develop a more NP-like phenotype than did mNP-CFU-F ( Fig. 1a ). 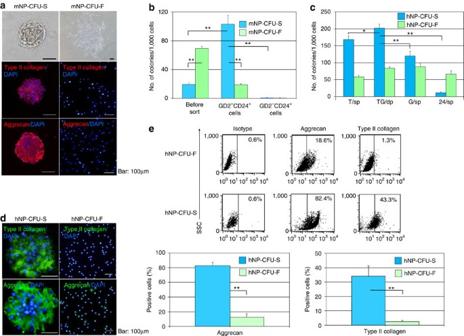Figure 1: Surface markers to select putative progenitor cells. (a) Two types of colonies derived from mouse primary NP cells in methylcellulose medium at 10 days (top panels): mNP-CFU-S (left) and mouse mNP-CFU-F (right). Immunocytochemical staining for the ECM indicates that mNP-CFU-S are robustly positive for type II collagen and aggrecan, whereas mNP-CFU-F are almost completely negative. Colonies were retrieved using 2 mM EDTA without enzymatic digestion and attached to slides using the Cytospin method. Scale bars, 100 μm. (b) One thousand mNP cells from each sorted population and unsorted cells were subjected to a CFA for 10 days. The frequency of mNP-CFU-S was higher in GD2+sorted cells than in unsorted mNP cells.n=5, **P<0.01 (ANOVA with Mann–WhitneyU-test). (c) One thousand human NP (hNP) cells from each sorted population were subjected to CFA for 10 days. The populations were Tie2+GD2–CD24–(Tie2 single-positive (T/sp) cells), Tie2+GD2+CD24–(Tie2 and GD2 double-positive (TG/dp) cells), Tie2–GD2+CD24–(GD2 single-positive (G/sp) cells) and Tie2–GD2–CD24+(CD24 single-positive (24/sp) cells). TG/dp cells had the greatest hNP-CFU-S formation among the four populations.n=5, *P<0.05, **P<0.01 (ANOVA with Mann–WhitneyU-test). (d) Comparison of ECM production between hNP-CFU-S and hNP-CFU-F. hNP-CFU-S were immunopositive for type II collagen and aggrecan, in contrast to the low expression in hNP-CFU-F. Scale bars, 50 μm. (e) Quantitative comparison of ECM production between hNP-CFU-S and hNP-CFU-F by flow cytometry. The cytoplasm of enzymatically dispersed and membrane-permeabilized cells from the colonies was stained. A higher percentage of immunopositive cells was detected in the cells from hNP-CFU-S than in those from hNP-CFU-F.n=3, **P<0.01 (ANOVA with Mann–WhitneyU-test). Data are represented as mean±s.d. DAPI, 4′,6-diamidino-2-phenylindole. Figure 1: Surface markers to select putative progenitor cells. ( a ) Two types of colonies derived from mouse primary NP cells in methylcellulose medium at 10 days (top panels): mNP-CFU-S (left) and mouse mNP-CFU-F (right). Immunocytochemical staining for the ECM indicates that mNP-CFU-S are robustly positive for type II collagen and aggrecan, whereas mNP-CFU-F are almost completely negative. Colonies were retrieved using 2 mM EDTA without enzymatic digestion and attached to slides using the Cytospin method. Scale bars, 100 μm. ( b ) One thousand mNP cells from each sorted population and unsorted cells were subjected to a CFA for 10 days. The frequency of mNP-CFU-S was higher in GD2 + sorted cells than in unsorted mNP cells. n =5, ** P <0.01 (ANOVA with Mann–Whitney U -test). ( c ) One thousand human NP (hNP) cells from each sorted population were subjected to CFA for 10 days. The populations were Tie2 + GD2 – CD24 – (Tie2 single-positive (T/sp) cells), Tie2 + GD2 + CD24 – (Tie2 and GD2 double-positive (TG/dp) cells), Tie2 – GD2 + CD24 – (GD2 single-positive (G/sp) cells) and Tie2 – GD2 – CD24 + (CD24 single-positive (24/sp) cells). TG/dp cells had the greatest hNP-CFU-S formation among the four populations. n =5, * P <0.05, ** P <0.01 (ANOVA with Mann–Whitney U -test). ( d ) Comparison of ECM production between hNP-CFU-S and hNP-CFU-F. hNP-CFU-S were immunopositive for type II collagen and aggrecan, in contrast to the low expression in hNP-CFU-F. Scale bars, 50 μm. ( e ) Quantitative comparison of ECM production between hNP-CFU-S and hNP-CFU-F by flow cytometry. The cytoplasm of enzymatically dispersed and membrane-permeabilized cells from the colonies was stained. A higher percentage of immunopositive cells was detected in the cells from hNP-CFU-S than in those from hNP-CFU-F. n =3, ** P <0.01 (ANOVA with Mann–Whitney U -test). Data are represented as mean±s.d. DAPI, 4′,6-diamidino-2-phenylindole. Full size image We then used a wide panel of antibodies to identify which cell surface markers correlated with the capability to form mNP-CFU-S (Methods). GD2 was identified as the most relevant marker. This disialoganglioside is a component of the plasma membrane found mainly in the nervous system and was identified recently as a marker for bone marrow mesenchymal stem cells (BM-MSC) [16] , [17] and umbilical cord mesenchymal stem cells [17] . As a number of GD2-expressing cells were also positive for CD24, we sorted GD2 + CD24 + mNP cells ( Supplementary Fig. S1 ) and confirmed that these cells generated mainly mNP-CFU-S, when seeded in the methylcellulose medium; the frequency increased from 19.6±2.8/1,000 in unsorted cells to 103.1±13.8/1,000 in sorted cells ( Fig. 1b ). GD2 positivity was also an indicator of proliferative capability on the plastic plates in ordinary liquid cultures ( Supplementary Fig. S1 ) because the GD2 – CD24 + population showed low growth and low capacity for mNP-CFU-S formation ( Supplementary Fig. S1 , Fig. 1b ). To find the precursor cells of these GD2 + cells, we investigated mouse primary cultures and identified a population expressing Tie2 that comprised Tie2 + GD2 – and Tie2 + GD2 + subpopulations. To understand the role of Tie2 + cells, we sorted Tie2 + GD2 – cells from day-10 cultured mNP cells and passaged them. After 10 days, 8.0±2.7% of the cells were Tie2 + GD2 + ( Supplementary Fig. S2 ). Thus, Tie2 + GD2 – cells were confirmed to be the precursor cells of Tie2 + GD2 + cells. Expansion of the cultures increased the percentage of Tie2 + GD2 + cells, which then disappeared by day 30, whereas the percentages of GD2 + CD24 + and GD2 – CD24 + cells increased ( Supplementary Fig. S3 ). In human NP cells, similar changes in the expression of Tie2, GD2 and CD24 were observed ( Supplementary Fig. S4 ). Sorted Tie2 + GD2 – cells from primary hNP cells generated Tie2 + GD2 + cells; on day 14, the Tie2 + GD2 + cell frequency was 14.5±5.6%. By contrast, sorted Tie2 – GD2 + cells generated neither Tie2 + GD2 – nor Tie2 + GD2 + cells ( Supplementary Fig. S5 ). These changes in the markers over time suggested a hierarchy originating from Tie2 + GD2 – CD24 – cells and followed in order by Tie2 + GD2 + CD24 – cells, Tie2 – GD2 + CD24 – cells and Tie2 – GD2 – CD24 + cells. To simplify the nomenclature, we henceforth refer to the hNP cell populations as follows: Tie2 + GD2 – CD24 – (Tie2 single-positive cells) as T/sp cells, Tie2 + GD2 + CD24 – (Tie2 and GD2 double-positive cells) as TG/dp cells, Tie2 – GD2 + CD24 – (GD2 single-positive cells) as G/sp cells and Tie2 – GD2 – CD24 + (CD24 single-positive cells) as 24/sp cells. To confirm the markers for purification of hNP progenitor cells, the following experiments were performed. First, we subjected TG/dp, G/sp and 24/sp cells to the CFA. As expected, TG/dp cells had the highest frequency of hNP-CFU-S formation (202.0±12.1/1000) among the three populations (G/sp: 120.0±14.3/1000, 24/sp: 11.4±2.8/1000) ( Fig. 1c ). Consistent with the results in the mouse, immunocytochemistry showed that hNP-CFU-S were positive for type II collagen and aggrecan, in marked contrast to hNP-CFU-F ( Fig. 1d ). ECM production was analysed quantitatively by immunofluorescence and flow cytometry ( Supplementary Methods ). The percentages of cells positive for collagen and aggrecan were higher in hNP-CFU-S (type II collagen: 34.3±6.9%, aggrecan: 82.4±4.9%) than in hNP-CFU-F (type II collagen: 0.9±0.1%, aggrecan: 12.1±4.9%) ( Fig. 1e ). Analysis of other stem cell markers indicated that CD271 expression was higher in T/sp and TG/dp cells (> 75% (addition of two populations expressing Tie2)) than in G/sp (<10%) or 24/sp (trace) cells. CD271 has been reported as a specific marker for human MSCs of diverse origin: from bone marrow [18] , [19] , adipose tissue [20] and synovial membranes [21] . Expression of Flt-1 was detected only in the T/sp and TG/dp cells. However, all populations were positive for CD44, CD49f, CD56, CD73, CD90, CD105 and CD166 ( Supplementary Fig. S6 ). These results support our proposed cellular hierarchy led by T/sp cells because T/sp and TG/dp cells were distinct from the two downstream G/sp and 24/sp populations; these results also confirm Tie2 and GD2 as markers. To assess whether harvested NP cells include migrated macrophage or cells from penetrated vasculature, we used flow cytometry to investigate the expression of markers of macrophages (CD45, CD14, CD11c), endothelial cells (CD31, CD34, CD144, Ulex europaeus Lectin, Von Willebrand Factor) and pericytes (CD146). We confirmed the lack of contamination by cells of haematopoietic or endothelial origin ( Supplementary Fig. S7 ), which was probably due to the precautions taken during sample collection (Methods). Single-cell-derived multipotent cells in TG/dp cells We predicted that progenitor cells were present within the population expressing Tie2 and performed the following experiments to verify their stem cell properties. However, because single T/sp cells did not proliferate enough for the study, TG/dp were used for clonal experiments. To demonstrate that hNP-CFU-S were derived from single cells, we inoculated single TG/dp cells separately into methylcellulose medium and confirmed the generation of hNP-CFU-S ( Fig. 2a ). 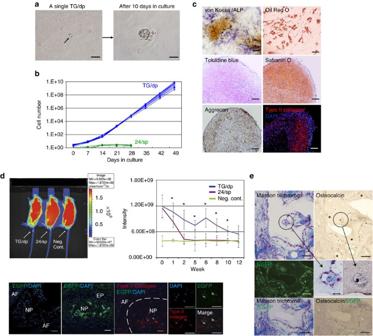Figure 2: Single-cell-derived multipotent cells in TG/dp cells. (a) Single TG/dp cells were purified from 7-day cultured hNP cells and inoculated into methylcellulose medium in 96-well culture plates. Single-cell-derived hNP-CFU-S were observed on day 10. (b) Population-doubling assays of TG/dp and 24/sp clones. TG/dp clones proliferated beyond 27 doublings, whereas 24/sp clones did not. (c) Clonal differentiation assays for mesenchymal lineages. Expanded clonal cultures from single TG/dp cells were cultured with induction medium for 21 days, and osteogenesis (von Kossa/ALP: Alkaline phosphatase), adipogenesis (Oil Red O) and chondrogenesis (toluidine blue, Safranin O, aggrecan and type II collagen) were detected. Scale bars, 100 μm. (d) Survival of the transplanted cellsin vivodetected by bioluminescence imaging (BLI). An EGFP-labelled TG/dp clone or EGFP-labelled 24/sp clone was injected into injured tail IVDs of NOD/SCID mice (1 × 105/IVD, respectively). BLI shows the survival of the TG/dp clone at day 31, whereas the 24/sp clone disappeared (upper left). Negative control mice without cell transplantation were used for calibration of autofluorescence. Superior survival of TG/dp cells is shown in the graph,n=3, *P<0.05, (ANOVA with Tukey’spost hoctest). EGFP-labelled TG/dp clone cells were detected inside the harvested disc sections (bottom left, mid-coronal; middle two panels, transverse sections). Coexpression of type II collagen with EGFP was detected by immunostaining (low magnification and high magnification, in three colours). Scale bars, 50 μm. (e) For osteogenesisin vivo, an EGFP-labelled TG/dp clone (1 × 105) was injected with a hydroxyapatite scaffold into a femoral bone defect model in NOD/SCID mice. Eight weeks later, Masson’s trichrome staining (top left) of the paraffin section identified blue collagenous fibres surrounding the EGFP+cells (bottom left). Immunohistochemical staining showed positive staining for osteocalcin (top right) and osteocalcin expression in the EGFP+cells (bottom right) in a cavity within the hydroxyapatite (*). Straight bars, 50 μm; arrowed bars, 20 μm, data are represented as mean±s.d. DAPI, 4′,6-diamidino-2-phenylindole; Neg. cont., negative control. Figure 2: Single-cell-derived multipotent cells in TG/dp cells. ( a ) Single TG/dp cells were purified from 7-day cultured hNP cells and inoculated into methylcellulose medium in 96-well culture plates. Single-cell-derived hNP-CFU-S were observed on day 10. ( b ) Population-doubling assays of TG/dp and 24/sp clones. TG/dp clones proliferated beyond 27 doublings, whereas 24/sp clones did not. ( c ) Clonal differentiation assays for mesenchymal lineages. Expanded clonal cultures from single TG/dp cells were cultured with induction medium for 21 days, and osteogenesis (von Kossa/ALP: Alkaline phosphatase), adipogenesis (Oil Red O) and chondrogenesis (toluidine blue, Safranin O, aggrecan and type II collagen) were detected. Scale bars, 100 μm. ( d ) Survival of the transplanted cells in vivo detected by bioluminescence imaging (BLI). An EGFP-labelled TG/dp clone or EGFP-labelled 24/sp clone was injected into injured tail IVDs of NOD/SCID mice (1 × 10 5 /IVD, respectively). BLI shows the survival of the TG/dp clone at day 31, whereas the 24/sp clone disappeared (upper left). Negative control mice without cell transplantation were used for calibration of autofluorescence. Superior survival of TG/dp cells is shown in the graph, n =3, * P <0.05, (ANOVA with Tukey’s post hoc test). EGFP-labelled TG/dp clone cells were detected inside the harvested disc sections (bottom left, mid-coronal; middle two panels, transverse sections). Coexpression of type II collagen with EGFP was detected by immunostaining (low magnification and high magnification, in three colours). Scale bars, 50 μm. ( e ) For osteogenesis in vivo , an EGFP-labelled TG/dp clone (1 × 10 5 ) was injected with a hydroxyapatite scaffold into a femoral bone defect model in NOD/SCID mice. Eight weeks later, Masson’s trichrome staining (top left) of the paraffin section identified blue collagenous fibres surrounding the EGFP + cells (bottom left). Immunohistochemical staining showed positive staining for osteocalcin (top right) and osteocalcin expression in the EGFP + cells (bottom right) in a cavity within the hydroxyapatite (*). Straight bars, 50 μm; arrowed bars, 20 μm, data are represented as mean±s.d. DAPI, 4′,6-diamidino-2-phenylindole; Neg. cont., negative control. Full size image The results of population-doubling assays started from single TG/dp or single 24/sp cells showed that the TG/dp clones had higher proliferative potential that expanded greatly beyond 27 cell doublings, whereas the 24/sp clones were markedly inferior ( Fig. 2b ). To evaluate their multipotent differentiation capability in vitro , TG/dp clonal cultures were subjected to 21 days of induction towards adipo-, osteo- or chondrogenesis ( Fig. 2c ). Nine of the 10 clones tested were bipotent (that is, could differentiate into two cell lineages) and four were tripotent (could differentiate into all three cell lineages). Thus, these clones were multipotent ( Table 1 ). To evaluate their potential in vivo , differentiation towards the NP and osteogenesis was assessed. Briefly, a TG/dp clone was transduced with the enhanced green fluorescent protein ( EGFP ) gene, and the cells were injected into injured tail IVDs of non-obese diabetic/severe combined immunodeficient (NOD/SCID) mice (1 × 10 5 /IVD). As a sham control, the same number (1 × 10 5 /IVD) of cells from a 24/sp clone was injected. Bioluminescence imaging was used to assess the survival and residence time of the implanted clones. Twelve weeks later, histological analysis of the harvested TG/dp clone-injected IVDs showed survival of EGFP + cells with an NP phenotype as detected by type II collagen coexpression, whereas the cells disappeared within 1–2 weeks in the sham control ( Fig. 2d ). To evaluate osteogenesis, an EGFP-labelled TG/dp clone (1 × 10 5 ) was injected together with a hydroxyapatite scaffold into a model femoral bone defect in NOD/SCID mice. Eight weeks later, healed bone was harvested and examined. Masson’s trichrome staining identified blue collagenous fibres surrounding EGFP + cells, which were also osteocalcin positive, as shown by immunostaining ( Fig. 2e ). Thus, the implanted TG/dp clone underwent histocompatible differentiation without prior induction in vitro . These results indicate that the TG/dp clones are multipotent. Table 1 Evaluation of the multipotency of TG/dp clones. Full size table Self-renewal capacity and NP tissue reorganization We performed serial cell transplantations to assess the abilities for self-renewal and NP tissue reorganization of TG/dp cells. Sorted hNP cells (1 × 10 5 ) transduced with the EGFP gene were transplanted subcutaneously with lethally irradiated (15 Gy) allogeneic hNP tissue (0.10 g) as a scaffold into five NOD/SCID mice, and the resulting tissues were harvested after 8 weeks ( Fig. 3a ). G/sp and 24/sp cells were used as controls. Only TG/dp achieved long-term engraftment in all recipients, and a number of labelled cells were detected in the transplants. By contrast, transplanted tissue scaffolds with or without control cells shrank markedly ( Fig. 3b , Supplementary Fig. S8 ). Histological analysis detected robust type II collagen and proteoglycan staining in the TG/dp transplants, indicating reorganization of NP tissue by TG/dp cells ( Fig. 3b ). Moreover, only TG/dp cells maintained the tissue weight at 0.11±0.03 g, in marked contrast to the decrease in the controls ( Fig. 3c ). Flow cytometry detected 29.0±9.3% labelled cells in the cells retrieved by enzymatic digestion from the TG/dp transplants, whereas only 4.4±3.8% were labelled in G/sp transplants and 0.5±0.4% in 24/sp transplants ( Fig. 3d , Supplementary Fig. S9 ). These results demonstrate the survival of TG/dp in vivo . 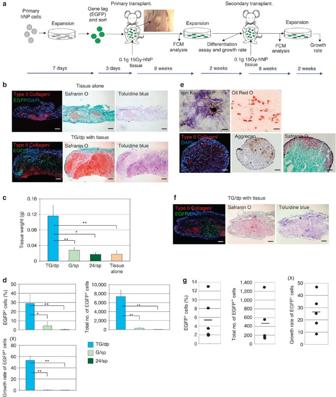Figure 3: Self-renewal capacity and NP tissue reorganization. (a) Strategy for testing the self-renewal capacity of TG/dp cells by serial subcutaneous transplantation into NOD/SCID mice. Sorted cell populations (TG/dp, G/sp and 24/sp cells) transduced with theEGFPgene were transplanted subcutaneously with lethally irradiated (15 Gy) allogeneic hNP tissues (0.10 g) as a scaffold. FCM, Flow cytometry. (b) Transplantation of scaffold tissue alone (upper panels). Transplantation of EGFP-labelled TG/dp cells (1 × 105) with tissue (lower panels). A number of EGFP+cells were detected in the TG/dp transplanted specimen, and histological analyses detected robust type II collagen and proteoglycan staining (Safranin O and toluidine blue). Scale bars, 200 μm. (c) Harvested tissue weight was maintained when transplanted with TG/dp. However, tissues transplanted without cells or with other cell populations (G/sp, 24/sp cells) lost considerable weight.n=5, **P<0.01 (ANOVA with Mann–WhitneyU-test). (d) Percentage of EGFP+cells detected by flow cytometry in cells retrieved from the transplants: 29.0±9.3% from TG/dp transplants, 4.4±3.8% from G/sp transplants and 0.5±0.4% from 24/sp transplants (top left). The corresponding cell numbers are shown (top right). After retrieval, the growth rates of cells cultured for 2 weeks were compared. The growth rate was higher in TG/dp transplants than in G/sp or 24/sp transplants (bottom left).n=5 *P<0.05, **P<0.01 (ANOVA with Mann–WhitneyU-test). (e) EGFP+cells from the TG/dp transplants maintained their multipotent differentiation ability towards osteogenesis (von Kossa/ALP), adipogenesis (Oil Red O) and chondrogenesis (type II collagen, aggrecan and Safranin O). Scale bars, 100 μm. (f) The expanded EGFP+cells from the primary TG/dp transplants were subjected to secondary transplantation with lethally irradiated (15 Gy) allogeneic hNP tissue (0.10 g) as a scaffold. EGFP+cells and type II collagen (left) and proteoglycan staining (Safranin O and toluidine blue, middle and right) were still detected in frozen sections of the harvested tissues. Scale bars, 200 μm. (g) The ratio and cell number of EGFP+cells retrieved from five individual recipients after secondary transplantation. EGFP-labelled TG/dp cells underwent two rounds of transplantation and still maintained high growth capacity for 2 weeks after retrieval. Data are represented as mean±s.d. Figure 3: Self-renewal capacity and NP tissue reorganization. ( a ) Strategy for testing the self-renewal capacity of TG/dp cells by serial subcutaneous transplantation into NOD/SCID mice. Sorted cell populations (TG/dp, G/sp and 24/sp cells) transduced with the EGFP gene were transplanted subcutaneously with lethally irradiated (15 Gy) allogeneic hNP tissues (0.10 g) as a scaffold. FCM, Flow cytometry. ( b ) Transplantation of scaffold tissue alone (upper panels). Transplantation of EGFP-labelled TG/dp cells (1 × 10 5 ) with tissue (lower panels). A number of EGFP + cells were detected in the TG/dp transplanted specimen, and histological analyses detected robust type II collagen and proteoglycan staining (Safranin O and toluidine blue). Scale bars, 200 μm. ( c ) Harvested tissue weight was maintained when transplanted with TG/dp. However, tissues transplanted without cells or with other cell populations (G/sp, 24/sp cells) lost considerable weight. n =5, ** P <0.01 (ANOVA with Mann–Whitney U -test). ( d ) Percentage of EGFP + cells detected by flow cytometry in cells retrieved from the transplants: 29.0±9.3% from TG/dp transplants, 4.4±3.8% from G/sp transplants and 0.5±0.4% from 24/sp transplants (top left). The corresponding cell numbers are shown (top right). After retrieval, the growth rates of cells cultured for 2 weeks were compared. The growth rate was higher in TG/dp transplants than in G/sp or 24/sp transplants (bottom left). n =5 * P <0.05, ** P <0.01 (ANOVA with Mann–Whitney U -test). ( e ) EGFP + cells from the TG/dp transplants maintained their multipotent differentiation ability towards osteogenesis (von Kossa/ALP), adipogenesis (Oil Red O) and chondrogenesis (type II collagen, aggrecan and Safranin O). Scale bars, 100 μm. ( f ) The expanded EGFP + cells from the primary TG/dp transplants were subjected to secondary transplantation with lethally irradiated (15 Gy) allogeneic hNP tissue (0.10 g) as a scaffold. EGFP + cells and type II collagen (left) and proteoglycan staining (Safranin O and toluidine blue, middle and right) were still detected in frozen sections of the harvested tissues. Scale bars, 200 μm. ( g ) The ratio and cell number of EGFP + cells retrieved from five individual recipients after secondary transplantation. EGFP-labelled TG/dp cells underwent two rounds of transplantation and still maintained high growth capacity for 2 weeks after retrieval. Data are represented as mean±s.d. Full size image Subsequently, the retrieved EGFP + cells from the TG/dp transplants were expanded and subjected to a mesenchymal lineage differentiation assay in vitro and to secondary transplantation. After primary transplantation and expansion, TG/dp maintained their tripotency in two of five recipients, and cells from all recipients showed bipotent capability ( Fig. 3e , Supplementary Table S1 ). Eight weeks after the secondary transplantation, 5.7±4.3% of the retrieved cells from five recipients were EGFP + and could still proliferate when passaged ( Fig. 3g , Supplementary Fig. S10 ). Histological analysis of the harvested transplants showed that they had been repopulated with labelled cells, which were surrounded by type II collagen and proteoglycan ( Fig. 3f ). These results suggest the existence of NP progenitor cells in the secondarily transplanted cells. Thus, only the multipotent cells in the TG/dp population that could differentiate into the three mesenchymal and NP lineages were self-renewing and, consequently, only they survived through the long-term xenograft trial. Function of Tie2–Ang-1 signalling in hNP In hNP tissue, Tie2 + NP cells coexpressing Ang-1, a ligand of Tie2, were detected by immunohistochemistry ( Fig. 4a ). We detected large amounts of Ang-1 in the supernatant of the NP cell cultures by enzyme-linked immunosorbent assay ( Supplementary Fig. S11 ). We added Tie2-blocking antibody to the serum-free culture medium and found that the number of apoptotic NP cells increased about twofold ( Fig. 4b ). This result suggested an innate anti-apoptotic effect of endogenous Ang-1 on hNP cells. We used real-time reverse transcription–polymerase chain reaction (RT–PCR) analysis to investigate the expression of Ang-1 mRNA in T/sp, TG/dp, G/sp and 24/sp cells. Gene expression in Tie2 – GD2 – CD24 – cells was used as a control. The expression of Ang-1 mRNA was lower in T/sp than in the other three populations ( Fig. 4c ), suggesting that the downstream TG/dp, G/sp and 24/sp populations supplied Ang-1 to T/sp. 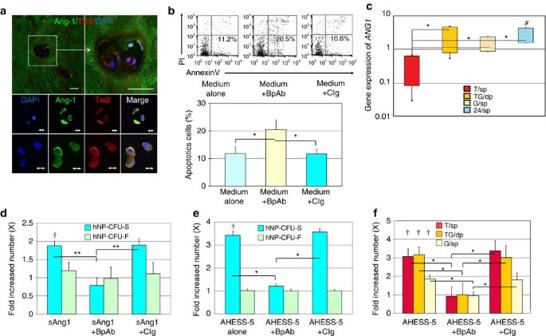Figure 4: Function of Tie2–Ang-1 signalling in the hNP. (a) In hNP tissues, immunohistochemistry detected Tie2+cells and Ang-1 expression in the matrix and cells (top left, cavities in hNP tissue; top right, the cavity magnified). Coexpression of Tie2 and Ang-1 was also detected (middle and bottom panels). Straight bars, 50 μm; arrowed bars, 10 μm. (b) Apoptosis assay in a serum-free culture of hNP cells. Addition of Tie2-blocking polyclonal antibody (BpAb) increased the number of apoptotic hNP cells after 48 h compared with medium alone or addition of goat control Ig (CIg). Apoptotic cells were identified by flow cytometry as Annexin V-positive and PI-negative cells.n=3, *P<0.05 (ANOVA with Mann–WhitneyU-test). (c) Quantitative comparison by real-time RT–PCR ofAng-1mRNA expression in the sorted hNP cell fractions. Gene expression levels were normalized to 18S rRNA and are presented relative to the levels in Tie2–GD2–CD24–cells.n=3, *P<0.05 between the sorted cell fractions, #P<0.05 compared with the Tie2–GD2–CD24–cell control (ANOVA with Mann–WhitneyU-test). (d) sAng1 significantly upregulated hNP-CFU-S generation. Note the significant reduction in hNP-CFU-S generation with addition of Tie2 BpAb compared with the CIg.n=5, **P<0.01, †P<0.05 compared with the no-sAng1 control (ANOVA with Mann–WhitneyU-test). (e) Cocultures in contact with AHESS-5 feeder cells through a culture insert (murine stromal cells overexpressing human Ang-1). The frequency of hNP-CFU-S increased significantly in the NP cells cocultured with AHESS-5, whereas the frequency of hNP-CFU-F did not change. Addition of Tie2 BpAb to the coculture medium blocked this effect.n=3, *P<0.05, †P<0.05 compared with the HESS-5 (without overexpression of Ang-1) control (ANOVA with Mann–WhitneyU-test). (f) A comparison of the three hNP cell populations (T/sp, TG/dp and G/sp) shows marked Ang-1-dependent growth in the two Tie2+populations (T/sp and TG/dp).n=3, *P<0.05 between the groups, †P<0.05 compared with the HESS-5 control. Data are represented as mean±s.d. Figure 4: Function of Tie2–Ang-1 signalling in the hNP. ( a ) In hNP tissues, immunohistochemistry detected Tie2 + cells and Ang-1 expression in the matrix and cells (top left, cavities in hNP tissue; top right, the cavity magnified). Coexpression of Tie2 and Ang-1 was also detected (middle and bottom panels). Straight bars, 50 μm; arrowed bars, 10 μm. ( b ) Apoptosis assay in a serum-free culture of hNP cells. Addition of Tie2-blocking polyclonal antibody (BpAb) increased the number of apoptotic hNP cells after 48 h compared with medium alone or addition of goat control Ig (CIg). Apoptotic cells were identified by flow cytometry as Annexin V-positive and PI-negative cells. n =3, * P <0.05 (ANOVA with Mann–Whitney U -test). ( c ) Quantitative comparison by real-time RT–PCR of Ang-1 mRNA expression in the sorted hNP cell fractions. Gene expression levels were normalized to 18S rRNA and are presented relative to the levels in Tie2 – GD2 – CD24 – cells. n =3, * P <0.05 between the sorted cell fractions, # P <0.05 compared with the Tie2 – GD2 – CD24 – cell control (ANOVA with Mann–Whitney U -test). ( d ) sAng1 significantly upregulated hNP-CFU-S generation. Note the significant reduction in hNP-CFU-S generation with addition of Tie2 BpAb compared with the CIg. n =5, ** P <0.01, † P <0.05 compared with the no-sAng1 control (ANOVA with Mann–Whitney U -test). ( e ) Cocultures in contact with AHESS-5 feeder cells through a culture insert (murine stromal cells overexpressing human Ang-1). The frequency of hNP-CFU-S increased significantly in the NP cells cocultured with AHESS-5, whereas the frequency of hNP-CFU-F did not change. Addition of Tie2 BpAb to the coculture medium blocked this effect. n =3, * P <0.05, † P <0.05 compared with the HESS-5 (without overexpression of Ang-1) control (ANOVA with Mann–Whitney U -test). ( f ) A comparison of the three hNP cell populations (T/sp, TG/dp and G/sp) shows marked Ang-1-dependent growth in the two Tie2 + populations (T/sp and TG/dp). n =3, * P <0.05 between the groups, † P <0.05 compared with the HESS-5 control. Data are represented as mean±s.d. Full size image We next used soluble human Ang-1 protein (sAng1) or coculture with feeder cells (murine stromal cells overexpressing human Ang-1 (AHESS-5)) [22] to demonstrate Ang-1-dependent upregulation of hNP-CFU-S generation and selective enhancement of proliferation of Tie2 + populations (T/sp, TG/dp). Culture with sAng1 increased hNP-CFU-S generation 1.9±0.1 times ( Fig. 4d ). Coculture with AHESS-5 increased generation of hNP-CFU-S 3.4±0.2 times ( Fig. 4e ) and proliferation of T/sp 3.1±0.4 times and TG/dp 3.2±0.4 times ( Fig. 4f ). All these effects were abolished completely by addition of Tie2-blocking antibody, thereby confirming the crucial role of Tie2–Ang-1 signalling in Tie2 + hNP cells. Expression of Tie2 and GD2 in IVD tissues To confirm the expression of Tie2 and GD2 in the IVD tissues, we stained mouse and human IVD tissues. Haematoxylin and eosin staining of the paraffin sections shows the histological profiles of mouse and human IVD tissues ( Fig. 5a ). Immunohistochemical staining detected both Tie2 and GD2 in cells in the NP area in mouse tail IVDs. Fixed IVD samples were frozen without decalcification and sectioned transversely. The locations of the marker molecules and the mNP cells are shown with phalloidin staining of F-actin in the cytoskeleton ( Fig. 5a ). We also identified these markers in frozen hNP sections. hNP cells stained positively with Tie2 or GD2 were detected clearly in the NP area in sections harvested from young donors ( Fig. 5b ). 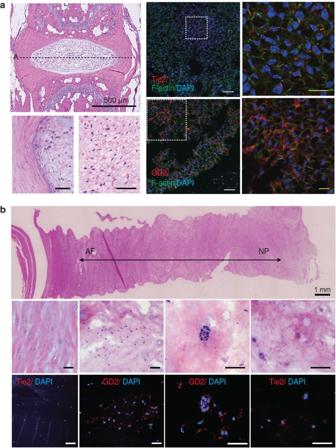Figure 5: Expression of Tie2 and GD2 in IVD tissues. (a) Histological analysis of paraffin sections of 9-week-old mouse tail IVDs sectioned in the mid-coronal plane and stained with haematoxylin and eosin (HE, top left). Line A indicates the direction of the sectioning, and the location was identified in the frozen sections used for immunofluorescence. The HE image on the far left shows the AF and NP border, and the right HE image shows the central NP. Fluorescent staining results show visualization of F-actin fibres of the cytoskeleton of mNP cells by phalloidin reagent (green). Expression of Tie2 (top middle, red in mNP cells; top right, the stained cells magnified) and GD2 (bottom middle, red in mNP cells; bottom right, stained cells magnified) on the cell surface was confirmed. Yellow scale bars, 20 μm; black and white bars, 50 μm. (b) Histological paraffin section of human IVD tissue (Thompson grade II) stained with HE identifies the corresponding locations in the following frozen sections indicated in the middle and lower panels (top panel; scale bar, 1 mm). Middle (HE) and bottom (immunofluorescence) panels of sections obtained from the AF (far left) to central NP (far right). No apparent immunostaining was detected for Tie2 or GD2 in the AF area (bottom left), but GD2+and Tie2+cells were detected (bottom centre to far right) in other areas. Scale bars, 50 μm. DAPI, 4′,6-diamidino-2-phenylindole. Figure 5: Expression of Tie2 and GD2 in IVD tissues. ( a ) Histological analysis of paraffin sections of 9-week-old mouse tail IVDs sectioned in the mid-coronal plane and stained with haematoxylin and eosin (HE, top left). Line A indicates the direction of the sectioning, and the location was identified in the frozen sections used for immunofluorescence. The HE image on the far left shows the AF and NP border, and the right HE image shows the central NP. Fluorescent staining results show visualization of F-actin fibres of the cytoskeleton of mNP cells by phalloidin reagent (green). Expression of Tie2 (top middle, red in mNP cells; top right, the stained cells magnified) and GD2 (bottom middle, red in mNP cells; bottom right, stained cells magnified) on the cell surface was confirmed. Yellow scale bars, 20 μm; black and white bars, 50 μm. ( b ) Histological paraffin section of human IVD tissue (Thompson grade II) stained with HE identifies the corresponding locations in the following frozen sections indicated in the middle and lower panels (top panel; scale bar, 1 mm). Middle (HE) and bottom (immunofluorescence) panels of sections obtained from the AF (far left) to central NP (far right). No apparent immunostaining was detected for Tie2 or GD2 in the AF area (bottom left), but GD2 + and Tie2 + cells were detected (bottom centre to far right) in other areas. Scale bars, 50 μm. DAPI, 4′,6-diamidino-2-phenylindole. Full size image Decrease of Tie2 + NP cells with ageing and degeneration To understand the clinical relevance of Tie2 + cells (T/sp and TG/dp cells), we analysed freshly dispersed hNP cells from surgical specimens with various degrees of IVD degeneration ( Supplementary Table S2 ). We found a large variation in the percentage of living cells that could be analysed after tissue digestion in relation to the donor’s age and the extent of degeneration. Therefore, we excluded propidium iodide (PI)-positive cells and analysed only the living cells using the live-gate system in flow cytometry (Methods). The frequency of Tie2 + (T/sp and TG/dp) cells and hNP-CFU-S in hNP cells decreased with the age of the donors ( Fig. 6a–c ). The decreases in Tie2 + (T/sp and TG/dp) cell frequency and hNP-CFU-S frequency correlated with the extent of disc degeneration ( Fig. 6d–f ) graded by morphology and magnetic resonance imaging. These data strongly suggest that exhaustion of the resources for regeneration may cause various changes within IVDs and support the relevance of Tie2 as a marker of NP progenitor cells. 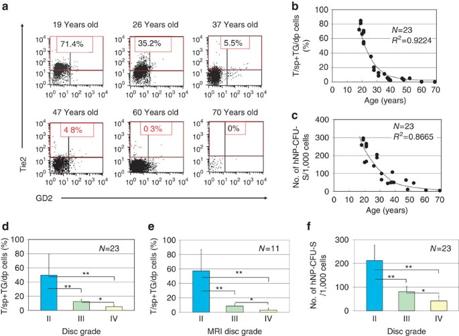Figure 6: Decrease of Tie2+NP cells with ageing and degeneration. hNP cells donated by patients were studied together with their clinical profiles. Cells were freshly dispersed and only cells detected by flow cytometry within the live and the PI-negative gate were analysed. (a) Representative flow cytometry data of Tie2 and GD2 cell positivity in different age groups. (b) The frequency of Tie2+cells (T/sp and TG/dp hNP cells) began to decrease before 20 years of age and correlated negatively with age (n=23,R2=0.9224). (c) The frequency of hNP-CFU-S generation also decreased with age (n=23,R2=0.8665). (d) The frequency of Tie2+cells (T/sp and TG/dp hNP cells) decreased in relation to the extent of disc degeneration graded by morphology and (e) with disc degeneration graded by diagnostic magnetic resonance imaging (n=11). (f) The frequency of hNP-CFU-S generation decreased in relation to the extent of disc degeneration graded by morphology (n=23). *P<0.05, **P<0.01 (ANOVA with Mann–WhitneyU-test). Data are represented as mean±s.d. Figure 6: Decrease of Tie2 + NP cells with ageing and degeneration. hNP cells donated by patients were studied together with their clinical profiles. Cells were freshly dispersed and only cells detected by flow cytometry within the live and the PI-negative gate were analysed. ( a ) Representative flow cytometry data of Tie2 and GD2 cell positivity in different age groups. ( b ) The frequency of Tie2 + cells (T/sp and TG/dp hNP cells) began to decrease before 20 years of age and correlated negatively with age ( n =23, R 2 =0.9224). ( c ) The frequency of hNP-CFU-S generation also decreased with age ( n =23, R 2 =0.8665). ( d ) The frequency of Tie2 + cells (T/sp and TG/dp hNP cells) decreased in relation to the extent of disc degeneration graded by morphology and ( e ) with disc degeneration graded by diagnostic magnetic resonance imaging ( n =11). ( f ) The frequency of hNP-CFU-S generation decreased in relation to the extent of disc degeneration graded by morphology ( n =23). * P <0.05, ** P <0.01 (ANOVA with Mann–Whitney U -test). Data are represented as mean±s.d. Full size image We have successfully identified NP progenitor cells in the Tie2 + and GD2 + populations from mouse and human IVDs. These cells were highly proliferative and were clonally capable of differentiating into multiple mesenchymal and NP lineages. Moreover, this multipotent ability was sustained through long-term engraftment and included the ability for self-renewal. IVD cells have been characterized poorly, which hinders the development of strategies for preventing and treating IVD degeneration. Cartilage chondrocytes have often been used as a reference for investigation of IVD cells. Chondrocytes are unique among non-transformed cells in that they are capable of anchorage-independent growth in soft agar [23] . In the current study, we found that NP cells could form clonal spheroid colonies in methylcellulose medium, and we used this characteristic to identify NP progenitor cells. We identified the recently reported BM-MSC marker GD2 [16] as a surface marker of NP-CFU-S. Although the exact mechanism explaining the difference between fibroblastic and spherical colony-forming cells is unclear, cell sorting with GD2 provided fundamental information about mouse and human NP cells. Our studies of GD2 + cells also led us to the discovery of their Tie2 + precursors. In addition to its expression in endothelial cells, Tie2 has been reported to be expressed in haematopoietic and neural stem cells, and is thought to regulate stem cell quiescence by promoting adhesion to the Tie2/Ang-1 stem cell niche [24] . The identification of the Tie2/Ang-1 system, which is usually associated with angiogenesis in the avascular IVD microenvironment, is surprising. However, NP cells have been reported to express vascular endothelial growth factor-A (VEGF-A) and its receptor, membrane-bound vascular endothelial growth factor receptor-1 (mbVEGFR-1) [25] . The investigators also showed that VEGF-A expression is promoted by hypoxic conditions and that this has an important role as a survival factor in the NP. As expression of Tie2/Ang-1 can be induced by local tissue hypoxia [26] , it is possible that the expression of Tie2/Ang-1 is induced in NP cells. Similar to the function of VEGF-A/mbVEGFR-1 in the resistance of the NP to apoptosis under hypoxic conditions, Tie2/Ang-1 signalling may have a role in NP cell maintenance and survival. CD24 has been reported as an NP-specific marker in the rat [27] . We found that in mNP cells, CD24 was associated with inferior proliferation in adhesive ordinary cultures and with low colony-forming capability in methylcellulose medium. These effects contrasted with those of GD2, which correlated with NP-CFU-S frequency and high proliferative capability ( Fig. 1b , Supplementary Fig. S1 ). In addition, Tie2 identified precursor cells that exhibited multipotency and self-renewal capacity. We also confirmed the expression of these three markers in hNP cells, which can be used to sort cells with different characteristics, as observed in the mouse. Thus, our newly identified markers, Tie2 and GD2, in combination with CD24, defined the irreversible cellular hierarchy in the mouse and human NP ( Fig. 7 ). 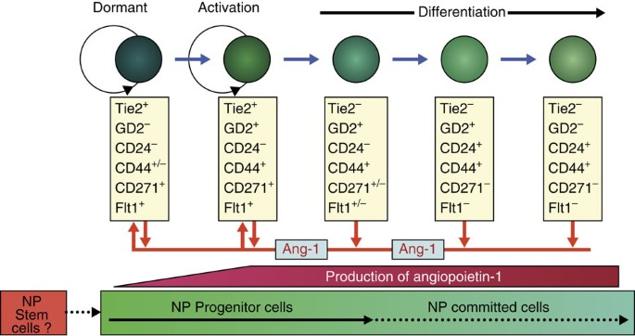Figure 7: Schematic model of NP cell differentiation. NP cell differentiation pathway was identified by cell surface markers based on experimental results. Individual surface marker expression is shown based on the experimental results (Supplementary Fig. S6). The arrowed circle indicates self-renewal; the blue arrows indicate irreversible change; the red arrows indicate supply of Ang-1 protein. Figure 7: Schematic model of NP cell differentiation. NP cell differentiation pathway was identified by cell surface markers based on experimental results. Individual surface marker expression is shown based on the experimental results ( Supplementary Fig. S6 ). The arrowed circle indicates self-renewal; the blue arrows indicate irreversible change; the red arrows indicate supply of Ang-1 protein. Full size image Among the populations of hNP cells sorted with these markers, T/sp and TG/dp cells were conspicuous by their expression of CD271. However, because of the limited proliferative ability of single T/sp cells, TG/dp cells were used for clonal experiments to verify their stem cell properties. As expected, when transplanted in vivo , TG/dp reorganized NP tissue and showed a high ECM-producing ability. In our previous study of xenografts using normal NP tissue from Lewis rats, implanted cells disappeared by 3 weeks [28] . This evidence demonstrates an immune response to subcutaneous xenografts even in the NOD/SCID mouse, and, accordingly, confirms the efficacy of TG/dp cells. The T/sp cells are currently the most primitive that have been identified and, because of their low proliferative ability, appear to be dormant ( Supplementary Fig. S4 ), although Tie2/Ang-1 signalling encourages these T/sp cells to proliferate in vitro . Therefore, T/sp cells might be identified if they could be expanded sufficiently without losing their properties. In clinical IVD specimens, more than 50% of the living cells from donors aged 18–21 years expressed Tie2, suggesting a large pool of progenitors. However, only a small proportion of these cells may be progenitor cells, and their clonal multipotency towards mesenchymal lineages was heterogeneous. Therefore, markers that are more restricted are needed to distinguish NP stem cells. Alternatively, these observations may be attributable to the quality of the NP tissues obtained from surgical specimens. Our specimens were not from healthy people, and the data should be interpreted carefully in association with the Thompson disc degeneration grading [29] and the Pfirrmann classification [30] . Surgically removed human NP tissues are mainly semi-fibrous except for gelatinous NP tissues from younger donors. In spite of the AF regions of the samples are more fibrous and show more lamellar formation than NP, the boundary between the NP and AF is obscure. To address this issue, we examined healthy mature mouse IVD tissues. In the mouse, the AF was well defined and could be protected from visible contamination to the NP in the samples collected for the in vitro experiments. Our immunohistochemical analysis showed the expression of the set of marker proteins in both the mouse and human NP. As in the mature mouse disc there is clear demarcation between AF and NP tissues, our results confirm the observation that progenitor cells are present in NP tissues. Both the flow cytometry and the histological analysis showed the presence of the same progenitor markers in hNP tissue as those found in the mNP. This is of interest because the cell population within the disc, especially in the NP, is reported to differ between species [31] . Our study shows for the first time an experimental model of NP differentiation induced from functional NP progenitor cells in vivo . Although further study is needed to elucidate the significance of Tie2 expression by NP cells, our data suggest that Tie2 is a sensitive marker of ageing and degeneration of IVDs, and will be a useful marker for the diagnosis of IVD degeneration. The effect of Tie2/Ang-1 signalling suggests that it has a niche function that could be a target for cytokine or gene therapy. Of the various biological therapies being tested, investigations of cell therapy have shown promising results in IVD degeneration treatment in animals [32] , [33] and have been extended recently to humans [34] , [35] . In subsequent iterations of such trials, we will test the ability of NP progenitor cells to induce tissue regeneration by delivering their resilient ECM-producing descendants. In addition, identifying the differentiation pathway of NP lineage cells will provide fundamental information for understanding IVD biology and informing therapeutic strategies. Mice Male C57BL/6 mice (CLEA Japan) were used for cell preparation, and male NOD/SCID mice (CLEA Japan) were used for in vivo transplantation. The animal experiments were approved by the Tokai University and were in accordance with the guidelines for the care and use of animals for scientific purposes at the Tokai University. Mouse NP tissues NP tissues from mouse tail IVDs were collected using a surgical microscope. hNP tissue specimens This study was approved by the Institutional Ethics Review Board of Tokai University School of Medicine. We obtained informed consent from the patients for the use of their IVD tissues. Twenty-three patients undergoing surgery for a burst fracture ( n =6), lumbar disc herniation ( n =14) or spondylolysis ( n =3) were enrolled in this study. The age of the patients ranged from 18 to 69 years, and tissue was evaluated with the Thompson grading system [29] and Pfirrmann classification system [30] . In cases of burst fracture where the upper end-plate was injured with a fractured vertebral body and the bottom end-plate was intact, we harvested the NP tissue from the disc attached to the intact bottom end-plate. In cases of grade III–IV discs, it was difficult to distinguish between the NP and inner AF, so we harvested the tissue from the central region of the NP. Cell isolation and culture hNP and mNP tissues were digested with TrypLE Express (Gibco) and then collagenase-P (Roche), washed twice with α-minimal essential medium (α-MEM; Gibco) and cultured in α-MEM supplemented with 10% fetal bovine serum (Cell Culture Bioscience). All cell culture was performed under hypoxic conditions of 5% O 2 and 5% CO 2 at 37 °C. The in vitro multidifferentiation potential of purified human NP cells was studied as described in Supplementary Methods . Colony-forming assay To assess colony formation, a single-cell suspension of 1.0 × 10 3 hNP or mNP cells was seeded into 35-mm diameter dishes and cultured in 1 ml of MethoCult H4230 methylcellulose medium (Stem Cell Technologies) for 10 days. Colonies (>10 cells) were counted using an inverted microscope. Identification of a marker to select colony-forming cells During the culture of primary mNP and hNP cells, 3 × 10 3 cells were collected every 3 days and subjected to the CFA. The frequency of spherical colonies was recorded. At the same time, changes in the expression of various cell surface markers on the cells were analysed by flow cytometry. Any marker that changed during the culture was recorded. Flow cytometry and cell sorting Cells were analysed using a FACSCalibur flow cytometer (BD Biosciences) and sorted using a FACS Vantage cell sorter (BD Biosciences). Only living cells were targeted by using a living (PI negative) gate except in the apoptosis assay. Cell cloning was also analysed using the FACSVantage cell sorter. The monoclonal antibodies used for analysis and purification are listed in Supplementary Methods . Histochemistry and immunohistochemistry Samples from human and mouse tissues and pellet cultures were fixed with 4% paraformaldehyde in phosphate buffer for 24 h. Frozen or paraffin sections were cut and stained as described in Supplementary Methods . Images were captured using an LSM510 12 META confocal microscope (Carl Zeiss) or an IX70 phase microscope (Olympus). In vivo transplantation One hundred thousand sorted and EGFP gene-transduced hNP cells were suspended in phosphate-buffered saline (100 μl) and injected subcutaneously into the flank area of NOD/SCID mice together with 15-Gy-irradiated 0.10-g hNP tissue (from a 21-year-old male donor not listed in Supplementary Table S2 ). Eight weeks after transplantation, the mice were killed under ether anaesthesia, and the subcutaneous human NP cell cysts were excised. Multipotent differentiation analysis in vivo One hundred thousand sorted and EGFP gene-transduced human NP cells were transplanted into injured tail IVDs and bone defects in mice as described in Supplementary Methods . Apoptosis assay To identify apoptosis in hNP cells, 10 μg ml −1 goat anti-Tie2-blocking polyclonal antibody (R&D Systems) or goat control Ig (R&D Systems) was added to the serum-free culture medium. After 48 h, the cells were stained with PI and fluorescein isothiocyanate-conjugated Annexin-V, according to the manufacturer’s instructions (Beckman Coulter). Real-time RT–PCR Cells were homogenized in lysis buffer, and total RNA was prepared using the RNAqueous Micro RNA isolation kit (Ambion, Applied Biosystems). mRNA was reverse transcribed using the High Capacity RNA-to-cDNA kit (Applied Biosystems). PCR analysis of the gene target was performed as described previously [36] . TaqMan gene expression assays (Applied Biosystems) were used as primers and probes. Statistical analysis Data are presented as the mean±s.d. Statistical significance was assessed by analysis of variance (ANOVA), and the Mann–Whitney U -test was used as a post hoc test. Significance was set as * P <0.05 and ** P <0.01 unless otherwise indicated. Correlations were analysed using the Spearman correlation coefficient. How to cite this article: Sakai, D. et al. Exhaustion of nucleus pulposus progenitor cells with ageing and degeneration of the intervertebral disc. Nat. Commun. 3:1264 doi: 10.1038/ncomms2226 (2012).